Brillouin cavity optomechanics with microfluidic devices Cavity optomechanics allows the parametric coupling of phonon- and photon-modes in microresonators and is presently investigated in a broad variety of solid-state systems. Optomechanics with superfluids has been proposed as a path towards ultra-low optical- and mechanical-dissipation. However, there have been no optomechanics experiments reported with non-solid phases of matter. Direct liquid immersion of optomechanics experiments is challenging, as the acoustic energy simply leaks out to the higher-impedance liquid surrounding the device. Here we confine liquids within hollow resonators to circumvent this issue and to enable optical excitation of mechanical whispering-gallery modes at frequencies ranging from 2 to 11,000 MHz. Our device enables optomechanical investigation with liquids, while light is conventionally coupled from the outer dry side of the capillary, and liquids are provided by means of a standard microfluidic inlet. Stimulated Brillouin scattering (SBS) [1] , [2] was considered for many years as an optical gain mechanism for lasers [3] and for nonlinear optics including phase conjugation [4] and slow light [5] . Subsequently, the platforms for Brillouin scattering were extended from bulk materials and fibres, to droplets [6] , nano-spheres [7] , photonic-crystal fibres [8] and crystalline resonators [9] , [10] . The recent demonstration of Brillouin scattering in microspheres [11] was followed by the Brillouin cooling [12] and excitation [10] , [13] of their vibrational modes as well; which indicates that Brillouin effects can serve as a general mechanism for actuating (and interrogating) vibration in various types of micro-mechanical resonators. In separate research on optofluidic devices [14] , [15] , the motion of liquids has been used to control light, but light has rarely been used to actuate a fluid [16] . In this study, we use the Brillouin scattering of light from sound to excite and measure vibration in a microfluidic optomechanical (μFOM) resonator. We design, fabricate and actuate μFOM resonators that exhibit mechanical deformation at their solid–fluid interface. Here confinement of the test fluid inside the device mitigates acoustic loss. Conversely, if an optomechanical resonator will just naively be submerged in a liquid, acoustic radiative losses will increase on account of the acoustic impedance of liquids being much larger than that of air. Experimental device and excitation mechanisms Our μFOM device ( Fig. 1a ) is fabricated from a lengthwise-drawn fused-silica capillary [17] with its radius modulated as a function of length (see Methods). At its widest point, this glass device forms a whispering-gallery mode (WGM) microresonator [18] that resonantly enhances both light and sound ( Fig. 1d ) while supporting a considerable overlap between the optical and mechanical modes. The acoustic modes are optically excited by means of forward [10] , [12] , [13] and backward [9] , [11] SBS, that is, F-SBS and B-SBS, respectively. 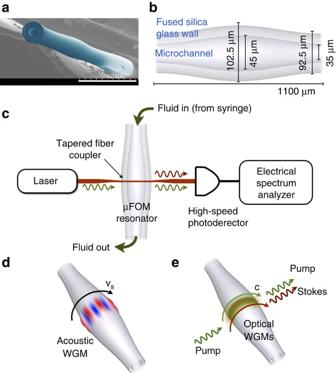Figure 1: Overview of the experiment. (a) Colourized scanning electron micrograph of a fused-silica μFOM device, showing the modulation of the radius as a function of position. Scale bar, 200 μm. (b) Dimensions of the device used to obtain mechanical WGM inFig. 3b–f. Not drawn to scale. (c) A tapered optical fibre is used to couple light in and out of the whispering-gallery optical modes of the μFOM resonator (without contact). We employ a telecom wavelength 1.5 μm pump laser without any modulation. A high-speed photodetector measures the mechanical vibration by means of its optical signature, that is, the beat note between the optical pump and the Stokes-scattered light. The experimental configuration for forward scattering is illustrated here. (d) Illustration of the mechanical WGMs on the μFOM resonator, showing that mechanical displacement is concentrated at the equator. The mode circulates at the velocity of sound,vs(e) Illustration of the optical WGMs of the μFOM resonator that travel at the speed of light,c. Figure 1: Overview of the experiment. ( a ) Colourized scanning electron micrograph of a fused-silica μFOM device, showing the modulation of the radius as a function of position. Scale bar, 200 μm. ( b ) Dimensions of the device used to obtain mechanical WGM in Fig. 3b–f . Not drawn to scale. ( c ) A tapered optical fibre is used to couple light in and out of the whispering-gallery optical modes of the μFOM resonator (without contact). We employ a telecom wavelength 1.5 μm pump laser without any modulation. A high-speed photodetector measures the mechanical vibration by means of its optical signature, that is, the beat note between the optical pump and the Stokes-scattered light. The experimental configuration for forward scattering is illustrated here. ( d ) Illustration of the mechanical WGMs on the μFOM resonator, showing that mechanical displacement is concentrated at the equator. The mode circulates at the velocity of sound, v s ( e ) Illustration of the optical WGMs of the μFOM resonator that travel at the speed of light, c . Full size image In the case of B-SBS [19] , the incoming pump light (frequency ω p ) photoelastically back-scatters from a high-frequency acoustic wave (frequency Ω) in the material to generate a lower frequency Stokes optical signal (frequency ω s =ω p −Ω) as shown in Fig. 2 . Simultaneously, electrostrictive pressure is generated by the two optical signals, which amplifies the acoustic wave. Optical spectrum analysis reveals the optical pump and Stokes signals, as shown previously in Tomes and Carmon [11] . The resulting beat note between pump and Stokes signals measured on an electrical spectrum analyser is representative of the high-frequency acoustic wave. This B-SBS-positive feedback process occurs near Ω=11 GHz mechanical frequency in silica when 1.5 μm pump light is used [19] . An experimental example of such a mode in this study is shown in Fig. 3f . 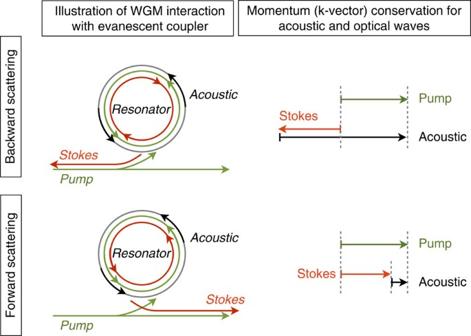Figure 2: Acoustic WGM frequencies are determined by momentum conservation. Conservation of momentum between photons and phonons dictates the acoustic WGM frequencies that are generated through SBS. Light travelling in the tapered waveguide evanescently couples to optical WGMs of the resonator, and is scattered to Stokes frequencies in either the forward or backward direction. In the case of back-scattering (B-SBS) momentum conservation enforces long acoustic k-vectors such that the acoustic modes are at high frequencies (that is, 10 GHz regime). Stokes light is received from the same tapered coupler in the backward direction. In forward scattering (F-SBS) momentum, conservation enforces that the acoustic modes are at much lower frequencies (that is, <1 GHz regime). Stokes light is received in the forward direction as illustrated inFig. 1c. Figure 2: Acoustic WGM frequencies are determined by momentum conservation. Conservation of momentum between photons and phonons dictates the acoustic WGM frequencies that are generated through SBS. Light travelling in the tapered waveguide evanescently couples to optical WGMs of the resonator, and is scattered to Stokes frequencies in either the forward or backward direction. In the case of back-scattering (B-SBS) momentum conservation enforces long acoustic k-vectors such that the acoustic modes are at high frequencies (that is, 10 GHz regime). Stokes light is received from the same tapered coupler in the backward direction. In forward scattering (F-SBS) momentum, conservation enforces that the acoustic modes are at much lower frequencies (that is, <1 GHz regime). Stokes light is received in the forward direction as illustrated in Fig. 1c . 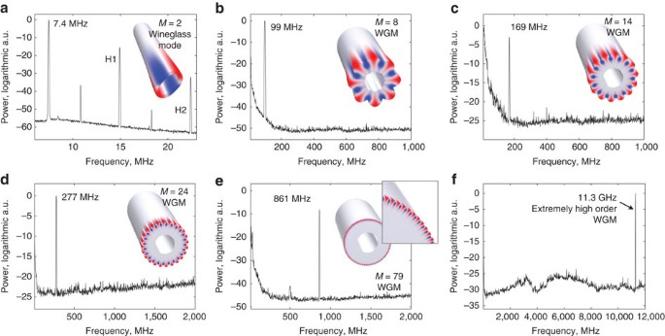Figure 3: Experimental observation of mechanical oscillations in water-filled devices. (a) Wineglass mechanical mode oscillation at 7.4 MHz. H1 and H2 are the first and second harmonics, respectively. Peaks at 10.81 and 18.27 MHz are caused by other mechanical modes of vibration being actuated. (b–e) Acoustic WGM oscillations of various azimuthal mode orders identified with the numberM. These modes are excited by forward SBS. (f) Extremely high-order acoustic WGM oscillations near 11 GHz are excited by backward SBS. a.u., arbitrary unit. Full size image Figure 3: Experimental observation of mechanical oscillations in water-filled devices. ( a ) Wineglass mechanical mode oscillation at 7.4 MHz. H1 and H2 are the first and second harmonics, respectively. Peaks at 10.81 and 18.27 MHz are caused by other mechanical modes of vibration being actuated. ( b – e ) Acoustic WGM oscillations of various azimuthal mode orders identified with the number M . These modes are excited by forward SBS. ( f ) Extremely high-order acoustic WGM oscillations near 11 GHz are excited by backward SBS. a.u., arbitrary unit. Full size image The case for forward scattering, that is, F-SBS, is identical to what is described above, except that the pump light photoelastically scatters in the forward direction such that the Stokes signal copropagates with the pump. This reversal of the scattering direction (to forwards) suggests that much smaller phonon momentum is required to bridge between the pump and Stokes momentum gap ( Fig. 2 ). As a result, lower acoustic frequencies (sub-GHz) are more likely for the F-SBS process. Additional details on the energy and momentum conservation requirements [20] for F-SBS and B-SBS in a circular resonator are discussed in [9] , [10] , [11] , [12] , [13] , [21] , [22] , [23] . Specifically for the capillary geometry that we use here, it is indicated [24] that a wide variety of acoustic WGMs exist in the shell-type geometry. Excitation of acoustic WGMs We experimentally excite acoustic WGM oscillations in a water-filled μFOM resonator, ranging in frequency from 99 to 11,000 MHz ( Fig. 3b–f ). As described in Fig. 2 , the ‘Brillouin’ optomechanical process [13] allows for excitation and measurement of these acoustic WGM oscillations by coupling continuous-in-time light at an optical resonance, while interrogating the optomechanical oscillation at the fibre output of the system (see Methods). No modulation of the pump laser is needed. We introduce and extract light from the optical WGMs by means of evanescent coupling with a tapered optical fibre [25] , [26] (as shown in Fig. 1c ). Optical ring-down measurements [27] indicate optical quality factors in excess of Q o =10 8 (highest measured Q o =1.6 × 10 8 ). No contact between the fibre and the μFOM resonator is required for mechanical transduction, so the acoustic quality factors are not degraded. The same optical fibre taper is used to extract the Stokes scattered light from the device, which is then used as a measure of the mechanical vibration within the structure [12] . All of our experiments are performed at room temperature and atmospheric pressure, and various solutions are introduced into the device by means of a syringe pump. We calculate the mechanical modes of the μFOM resonator using three-dimentional finite element modelling using Comsol Multiphysics ( http://www.comsol.com/ ) as described previously in Zehnpfennig et al . [22] and Bahl et al . [24] Only the glass capillary is modelled, without a liquid, to extract the mechanical modes of the device that correspond to the observed oscillation. Each of these modes is identified with a M-number which is the azimuthal mode order quantifying the number of acoustic wavelengths around the equatorial circumference of the device. In addition, a M =2 WGM at 7 MHz is observed ( Fig. 3a ), that is generally referred to as a wineglass mode. The harmonics in this wineglass mode oscillation (H1, H2 in Fig. 3a ) are typical for such low frequency modes and result from the fact that this is a standing-wave type vibration excited by centrifugal radiation pressure [28] , [29] , [30] , [31] , as opposed to the travelling-wave vibrations in Fig. 3b–f . Quantifying solid–liquid interaction The penetration of sound to the liquid scales with the ratio between the acoustic wavelength and the thickness of the resonator wall. Therefore, the 7.4 MHz (M=2) mode is calculated to have large penetration into the fluid ( Fig. 4a ). Finite element calculation shows that the 99 MHz (M=8) mode has a 16% penetration to fluid, defined by the deformation amplitude at the inner fluid interface divided by the maximum deformation ( Fig. 4b ). An arguably better method of quantifying the efficiency of interaction with the liquid would be to calculate the ratio of energy stored in fluid deformation to the energy stored in the glass deformation. As this requires modelling of the fluid as well, this preferred quantification method is not chosen here. The higher M modes have lower penetration into the liquid. However, as we can fabricate the resonator with walls as thin as 560 nm (ref. 32 ) we believe that a large acoustic penetration to water will be possible in such thin-wall silica bubble resonators even for the 11 GHz mode ( M ≈650), which can open a rare hypersonic window for the acoustic analysis of liquids. Reduction in wall thickness may even allow access to an interesting regime where giant-enhanced Brillouin scattering is predicted [33] . 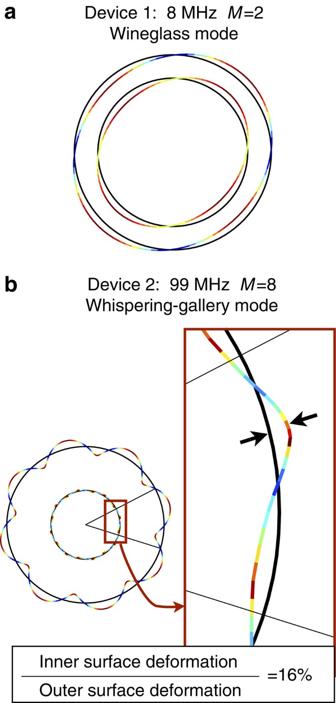Figure 4: Calculated equatorial mechanical mode profiles. (a) For theM=2 wineglass mode at 8 MHz (experimentally appears at 7.4 MHz, seeFig. 3a) the displacement ratio of internal and external surfaces is almost 1:1 at the equator. (b) For the experimentally observedM=8 acoustic WGM at 99 MHz (seeFig. 3b), the inner surface experiences 16% displacement relative to the outer surface. Figure 4: Calculated equatorial mechanical mode profiles. ( a ) For the M =2 wineglass mode at 8 MHz (experimentally appears at 7.4 MHz, see Fig. 3a ) the displacement ratio of internal and external surfaces is almost 1:1 at the equator. ( b ) For the experimentally observed M =8 acoustic WGM at 99 MHz (see Fig. 3b ), the inner surface experiences 16% displacement relative to the outer surface. Full size image Characterization of mechanical mode We measure that the minimum power required to excite these oscillations in the water-filled μFOM device is 158 μW ( Fig. 5a ). We also measured a mechanical quality factor Q m =4,700 for the 99 MHz ( M =8) mode in this water-filled device ( Fig. 5b ), via the sub-threshold oscillation linewidth, which implies Q m × Frequency =4.6 × 10 11 . This ‘f-Q product’ compares well against the previously measured Q m =12,300 in a solid silica sphere for a 95-MHz mode [12] . 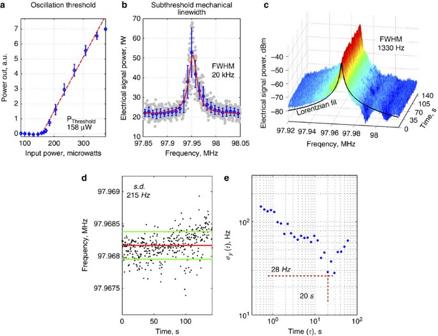Figure 5: Characterization of 99 MHz acoustic WGM in a water-filled device. (a) Lowest observed optical threshold power to excite mechanical oscillation is 158 μW. Error bars indicate variance of each averaged measurement. (b) The intrinsic mechanical linewidth (mechanical quality factor) is directly observed at very low input optical power. Error bars indicate local variance of the averaged raw data. (c) A spectrogram of the mechanical oscillation frequency spectrum is obtained with above-threshold input optical power.xaxis is mechanical frequency measured through the beat note of the pump and the vibration-scattered Stokes light on a photodetector,yaxis is logarithmic mechanical oscillation power, and depth axis is time. In this example, the laser was rapidly scanned back-and-forth through the region of the optical mode that exhibits phase-matching for this mechanical oscillation. (d) Peak frequencies extracted from spectrogram ofcshow a s.d. of 215 Hz. (e) Allan deviation plot of the frequency data indprovides an estimate of the potential sensor resolution. a.u., arbitrary unit. Figure 5: Characterization of 99 MHz acoustic WGM in a water-filled device. ( a ) Lowest observed optical threshold power to excite mechanical oscillation is 158 μW. Error bars indicate variance of each averaged measurement. ( b ) The intrinsic mechanical linewidth (mechanical quality factor) is directly observed at very low input optical power. Error bars indicate local variance of the averaged raw data. ( c ) A spectrogram of the mechanical oscillation frequency spectrum is obtained with above-threshold input optical power. x axis is mechanical frequency measured through the beat note of the pump and the vibration-scattered Stokes light on a photodetector, y axis is logarithmic mechanical oscillation power, and depth axis is time. In this example, the laser was rapidly scanned back-and-forth through the region of the optical mode that exhibits phase-matching for this mechanical oscillation. ( d ) Peak frequencies extracted from spectrogram of c show a s.d. of 215 Hz. ( e ) Allan deviation plot of the frequency data in d provides an estimate of the potential sensor resolution. a.u., arbitrary unit. Full size image This 99 MHz ( M =8) mode of vibration can be maintained as long as the CW input laser power is provided. A spectrogram demonstrating this stability ( Fig. 5c ) is obtained over 140 seconds while periodically scanning through the optical resonance that excites this mechanical mode. While such oscillation data is typically captured with the laser at a fixed frequency, we practically found that scanning our pump laser through the optical resonance is more repeatable. This is because scanning is less affected by unknown drifts. We detect the peak oscillation frequencies ( Fig. 5d ) in this spectrogram by means of Lorentzian curve fits ( Fig. 5c ) at each time-point. The standard deviation of the peak frequency is calculated to be 215 Hz along this 140-second period. In order to better characterize the stability of the oscillation and the ability of this system to function as a sensor, we calculate the Allan deviation (square root of the two-point variance) of the frequency data, which charts the frequency deviation as a function of averaging time ( Fig. 5e ). It is seen that short-term and long-term frequency drifts dominate device performance. For instance, the long-term upward drift in Fig. 5d manifests as an up-turn in the Allan Deviation data ( Fig. 5e ) for long averaging times. The short-term frequency instabilities manifest as a large deviation for short averaging times. A ‘sweet spot’ occurs in between, indicating that a 20-s moving average of the sensor output will give us best resolution. Operation with high-density high-viscosity liquids We perform an experiment to prove that the optomechanical interaction can be sustained even when the motional mass is high (that is, high-density liquid) and when the fluid-related acoustic energy losses are high (that is, high viscosity). We incorporate sucrose (table sugar) into an aqueous solution inside the resonator and measure the sensitivity of the optomechanically actuated wineglass mode to the sucrose concentration of the fluid. Optomechanical oscillation is observed at all tested sucrose concentrations. The resulting relationship between acoustic frequency and the sucrose concentration exhibits a non-monotonic trend, which we plot in Fig. 6 along with a linear fit to the data. The net decreasing frequency trend is consistent with increasing effective mass of the oscillator as the fluid density increases. The visibly non-monotonic nature of the trend, however, might originate from non-perturbative high-sugar concentrations resulting in nonlinear change in frequency. For a complete model one should consider the change in the fluid properties with the sucrose concentration, including the change of speed of sound [34] . We note that at the highest sucrose concentration that we test in this experiment, the solution has a viscosity that is ~3-times greater than that of blood [35] . The actuation of optomechanical oscillation with such a high-viscosity liquid opens up the possibility for investigating the acoustic properties of viscous bio-analytes. 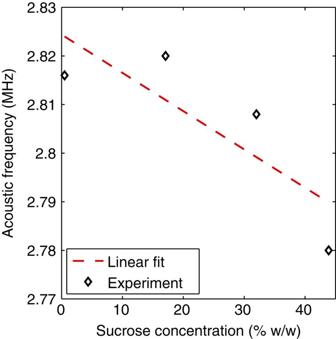Figure 6: Optomechanical sensing of sucrose solutions. We experimentally measure the frequency of a 2.8 MHz wineglass acoustic mode (M=2) as the concentration of sucrose solution inside the μFOM resonator is varied. The size of the markers in the figure is approximately the s.d. (better than 1 kHz) of each frequency measurement. The dashed red line is a linear fit to the data, which indicates a downward trend consistent with increasing effective mass of the resonator. Resonator outer diameter is 184 μm. Figure 6: Optomechanical sensing of sucrose solutions. We experimentally measure the frequency of a 2.8 MHz wineglass acoustic mode ( M =2) as the concentration of sucrose solution inside the μFOM resonator is varied. The size of the markers in the figure is approximately the s.d. (better than 1 kHz) of each frequency measurement. The dashed red line is a linear fit to the data, which indicates a downward trend consistent with increasing effective mass of the resonator. Resonator outer diameter is 184 μm. Full size image In this work, we demonstrate a bridge between optomechanics and microfluidics by confining various liquids inside a hollow microfluidic optomechanical resonator. We present experimental evidence that the optomechanical interaction in the μFOM device is dependent on the fluid contained within. These results are, therefore, a step towards novel experiments probing optomechanics on non-solid phases of matter. In particular, the high frequency, high quality-factor mechanical modes demonstrated in this work may enable strongly localized, high-sensitivity, optomechanical interaction with chemical and biological analytes [36] , [37] as environmental parameters like pressure and cell nutrients are relatively easy to control inside the hollow resonator [32] , [38] , [39] , and as the liquid volume within the device is the scale of a living cell. In contrast to other optomechanical systems that typically involve standing-wave mechanical vibrations, here circulating phonons comprises the acoustic WGMs [13] , [22] , which are essentially acoustic vortices [40] , [41] , [42] . These travelling-wave type acoustic modes carry angular momentum, which creates possibility of using μFOM devices to enable optomechanical interactions with vortices in various liquids [43] , [44] , [45] and condensates. Microfluidic device fabrication The μFOM device ( Fig. 1a ) is fabricated with a fused-silica glass capillary that is pulled lengthwise using linear actuators, while being heated with infrared lasers (CO 2 at 10.6 μm). By controlling the power of the manufacturing laser in the process of pulling, we can control the device diameter along its length. This process has also previously been developed in Sun et al . [17] Optical WGMs and acoustic WGMs are simultaneously well-confined in the regions of large diameter sandwiched between regions of narrow diameter ( Fig. 1d ), enabling a high-degree of modal overlap. Therefore, these large diameter regions form the μFOM resonators, and multiple such resonators can be built on a single capillary. Experimental method The μFOM resonator is placed in close proximity (<1 μm distance) to tapered optical fibre [25] , [26] (as shown in Fig. 1c ), such that evanescent coupling from the taper allows light to be introduced and extracted from the optical WGMs of the device. A CW fibre-coupled tunable 1.5 μm laser is used as the source (Newfocus TLB-6328), and a fibre-coupled high-speed photodetector is used to monitor vibration. Mechanical vibration is stimulated within the device by pumping-specific optical resonances where the three-mode phase-match exists. The internally generated Stokes-shifted laser is then also collected by the tapered fibre, and the temporal interference of this new Brillouin laser against the partially transmitted pump laser is used to infer the mechanical response using the photodetector [12] , [13] . An optical spectrum analyser is used to verify that four-wave mixing and Raman scattering are not responsible for the beat note observed in the electrical spectrum. How to cite this article: Bahl, G. et al . Brillouin cavity optomechanics with microfluidic devices. Nat. Commun. 4:1994 doi: 10.1038/ncomms2994 (2013).